CRISPR-Cas and restriction–modification systems are compatible and increase phage resistance Bacteria have developed a set of barriers to protect themselves against invaders such as phage and plasmid nucleic acids. Different prokaryotic defence systems exist and at least two of them directly target the incoming DNA: restriction–modification (R-M) and CRISPR-Cas systems. On their own, they are imperfect barriers to invasion by foreign DNA. Here, we show that R-M and CRISPR-Cas systems are compatible and act together to increase the overall phage resistance of a bacterial cell by cleaving their respective target sites. Furthermore, we show that the specific methylation of phage DNA does not impair CRISPR-Cas acquisition or interference activities. Taken altogether, both mechanisms can be leveraged to decrease phage contaminations in processes relying on bacterial growth and/or fermentation. For bacteria, phages are arguably the most challenging enemies found in their environments. Not only do phages represent the most abundant biological entities on our planet (estimated at 10 31 phages) [1] , they are also highly diversified due to their genome plasticity. The most studied phages have double-stranded DNA (dsDNA) genome encapsidated in a protein capsid, which is connected to a tail [2] . To shield against these invading viruses, bacteria have evolved and perfected a plethora of defence mechanisms [3] . Among them, two systems act by specifically cleaving the incoming viral DNA as it enters the host cells, namely the restriction–modification systems (R-M) and the CRISPR-Cas systems (Clustered Regularly Interspaced Short Palindromic Repeats loci, coupled to CRISPR-associated genes). R-M systems are almost universal and they have been found in ~90% bacterial and archaeal genomes [4] . These systems are well known, exhaustively studied, and their activities have been exploited for decades, particularly in genetic engineering. In general, within a cell, a methyltransferase protects host DNA by modifying specific nucleic acid. The restriction endonuclease cleaves any foreign DNA containing a specific recognition site, which has not previously been protected by the same modification [3] . The incoming DNA is usually restricted before the methylation occurs, and, the more a phage genome contains restriction sites, the more susceptible it is to restriction [5] , [6] . On the other hand, a phage genome with methylated restriction sites (or without these specific sites) will no longer be cleaved by the endonuclease activity and the phage infection will proceed, leading to cell death and to the release of new virions. R-M systems have been classified into four main types [7] , with type II systems being the best known and widely used in molecular biology. These enzymes cleave inside or close to the recognition site to produce 5′-P or 3′-OH extremities. CRISPR-Cas systems are found in roughly half of sequenced bacterial genomes and over 80% of archaeal ones [8] . They consist of a CRISPR locus composed of direct repeats separated by short stretches of variable DNA called spacers. Various cas ( CRISPR-associated ) genes are often flanking the CRISPR array [9] . Overall, these systems encode operons possessing extraordinarily diverse architectures for both the cas genes and the spacers content. CRISPR-Cas systems are currently classified into three major types (I, II and III), divided into several subtypes [10] . To provide immunity, this system follows at least three general recognized steps: acquisition, biogenesis of small RNAs and interference. In the acquisition step, a new repeat-spacer unit is added to the CRISPR locus, in which the spacer is acquired from a part of the invading DNA (named the protospacer) often through the involvement of PAM sequences (protospacer-adjacent motif) [11] , [12] . A CRISPR transcript is then produced and cleaved within the repeats by Cas protein(s), with or without the help of other host proteins, to produce smaller RNAs (crRNA). In the interference step, these small mature crRNAs and Cas proteins guide and cleave in a sequence-specific manner the invading DNA to ensure cell defence. Phages can successfully infect a strain carrying a CRISPR-Cas system if its genome does not carry the matching protospacer or if the latter is mutated [12] , [13] . CRISPR-Cas type II systems have been considerably studied because they offer practical applications in generating phage-resistant strains and in genome editing [14] , [15] , [16] , [17] , [18] , [19] , [20] , [21] and the three main steps have been experimentally confirmed [22] . Recent bioinformatic analyses showed that genes encoding phage defence system components in bacterial and archaea typically cluster in defence islands [23] . These analyses suggested that some of these defence mechanisms, including CRISPR-Cas and R-M, might be functionally coupled [24] . On the other hand, they may also work independently or interfere with each other. Here, we experimentally investigate the faith of phage infection on a bacteria cell having both functioning CRISPR-Cas and R-M systems. Both systems are shown to be compatible, cleave the invading DNA and provide bacteria with increased phage resistance. We also show that the CRISPR-Cas system is able to cleave phage DNA previously methylated by the R-M system. The use of two different defence strategies could help tip the balance in bacterial favour in this co-evolutionary arm race against virulent phages. Combinations of bacterial defence systems We used Streptococcus thermophilus as a bacterial model because its CRISPR-Cas systems have been shown previously to be highly active in strain DGCC7710 (refs 12 , 25 , 26 , 27 ) and its mode of action (adaptation, biogenesis of crRNA and interference) has arguably been the most studied. This wild-type S. thermophilus strain is sensitive to several virulent phages including the model phage 2972 (ref. 28 ). This particular bacterial strain also carries two type II CRISPR-Cas systems (CR1 and CR3) and both can acquire new spacers during a phage challenge, rendering these derivatives phage-resistant (called CRISPR-BIMs, for bacteriophage-insensitive mutants) [13] , [27] . 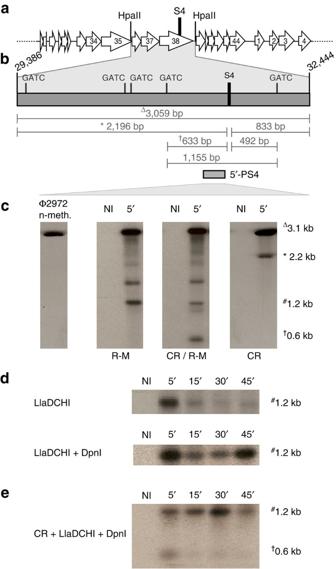Figure 1: R-M and CRISPR1-Cas system cleave phage DNA. (a) Region of the phage 2972 genome analysed in this study. Each arrow represents an open reading frame (ORF) previously annotated28. The positions of protospacer S4 as well as HpaII restriction sites (5′-CCGG-3′) are indicated. (b) Zoom on a specific HpaII fragment of phage 2972 genome. LlaDCHI and DpnI restriction sites (5′-GATC-3′) are indicated. Details of expected cleaved and detected fragments by Southern hybridizations are given below, and the rectangle is a schematic representation of the probe used (5′-PS4) for hybridizations. (c–e) Southern hybridization of phage-infectedS. thermophilusstrains using wild-type phage 2972. Samples were taken after 5 min or after 15, 30 and 45 min intervals following the addition of phages.S. thermophilusstrains DGCC7710+R-M, CRISPR-BIM S4, and BIM S4+R-M are represented by R-M, CRISPR-Cas (CR), and both respectively. The expected and detected cleaved DNA fragments are specified using different symbols (Δ, *, † and #). Five to ten micrograms of total DNA from DGCC7710 and CRISPR-BIM S4 were loaded per lane. All fragments belong to a different combination of CRISPR and/or R-M cleavage sites, but only the more important fragments implicating the CRISPR site are detailed inb. (c) Phage genome cleavage inS. thermophilusstrains. The first panel to the left indicates the positive control (phage 2972 DNA). Specific cleavage activities detected ina: (i) R-M+strain (second panel; shorter fragment of ~1.2 kb), (ii) CRISPR-Cas strain (BIM S4, fourth panel; fragment of ~2.2 kb), (iii) strain carrying both an active R-M and CRISPR-Cas systems (third panel; shorter fragment of ~0.6 kb). (d) The 1.2-kb fragment obtained inc(second panel) in phage-infectedS. thermophilusstrain DGCC7710 carrying the LlaDCHI R-M system was followed over time (LlaDCHI; upper panel) in Southern hybridization assays. The same infected samples were restricted with DpnI, which cleaves only when its recognition site (5′-Gm6ATC-3′) is methylated (LlaDCHI+DpnI; lower panel). (e) The smaller fragment (0.6 kb) obtained inc(third panel) in phage-infectedS. thermophilusstrain DGCC7710 CRISPR-BIM S4 was followed over time. Only DpnI-restricted samples are shown as they give the same results as with LlaDCHI alone. The acquisition of one matching spacer to phage 2972 genome into DGCC7710 CR1 spacer array provides resistance against this virulent phage at an efficiency of plaquing (EOP) of 10 −6 ( Table 1 ). The interference is due to the rapid cleavage of the invading viral dsDNA in the targeted protospacer, 3 bp upstream the PAM extremity [26] , [27] . Table 1 Effects of CRISPR-Cas and R-M systems on phage 2972 infectivity. Full size table Even though a type I R-M has been detected in the strain DGCC7710 (ref. 29 ), no restriction activity could be shown in vivo and in vitro . In fact, overall S. thermophilus R-M systems have been poorly studied [30] , [31] , [32] , [33] ( Table 2 ). Thus, to verify whether CRISPR-Cas system can be combined with a R-M system to increase the overall phage defence, we elected to introduce plasmid pSRQ707 into the strain DGCC7710 ( Table 3 ). This plasmid contains the genes coding for the LlaDCHI R-M system of Lactococcus lactis [34] , and was previously shown to be active and conferring phage resistance in S. thermophilus [35] . L. lactis is another lactic acid bacterium found in the same phage-containing ecological niche (milk) as S. thermophilus . LlaDCHI belongs to the type II restriction enzyme DpnII family, as it specifically recognizes the double-stranded unmethylated sequence 5′-GATC-3′. LlaDCHI system possesses a restriction endonuclease (LlaDCHI-C), a Dam-like methylase (LlaDCHI-A, for adenine methylation of dsDNA) [36] , and a second methyltransferase (LlaDCHI-B), homologous to DpnA (from DpnII system), thought to methylate single-stranded DNA [34] , [37] , [38] . Table 2 S. thermophilus native R-M system and phage resistance. Full size table Table 3 Characteristics of bacterial strains used in this study. Full size table The addition of LlaDCHI into S. thermophilus DGCC7710 (RM-BIM), without any CRISPR interference (i.e., no active targeting spacer against phage 2972), provides a resistance against virulent phage 2972 at an EOP of 10 −5 ( Table 1 ). This level of phage protection is similar to what is observed with a CRISPR-BIM carrying one targeting spacer ( Table 1 ). Unexpectedly, this similar level of resistance is obtained despite a significant difference in the number of targets. While the CRISPR-Cas system targets the only selected protospacer in the genome of 2972, the endonuclease LlaDCHI can target 35 different GATC sites on the same genome. It has been suggested previously that the number of restriction sites is correlated with the phage resistance level, specifically a high number of restriction sites in a phage genome usually leads to a decreased ability to replicate on a RM-BIM [6] . These data either suggest that the CRISPR-Cas system efficiently cleaves phage DNA to block its replication, that the methylase activity of the R-M system efficiently modifies phage DNA to allow replication, or that both are in play. To determine the compatibility for the two defence mechanisms, the same R-M system was also introduced into the previously characterized CRISPR-BIM, namely S4 (ref. 12 ). When combined, the two systems reduced phage infectivity under the limit of detection, which was less than an EOP of 10 −9 , in the conditions employed. This indicates that both systems are compatible, and their combination represents a very high level of protection against genetic invaders. DNA cleavage activities Within the phage-infected bacterial cell, as soon as the endonuclease (R) and the CRISPR-Cas systems find their incoming phage target (non-methylated recognition sites or matching protospacer sequence, respectively), both systems will cleave the dsDNA phage genome, thereby blocking phage replication. We followed the dsDNA cleavage activity of both systems by Southern hybridizations during a phage time-course infection. Total DNA (bacterial and phage) was isolated from various phage-infected cells at time intervals and then digested in vitro with HpaII to facilitate gel migration and subsequent analyses. Considering that the 34.7-kb genome of 2972 contains 35 GATC sites, only the fate of an ~3.1-kb HpaII fragment was followed here using specific probes ( Fig. 1a ). This selected 3.1-kb fragment contains 5 GATC sites as well as the targeted protospacer S4. Theoretical cleavage sites that are possible within this 3.1-kb fragment are illustrated in Fig. 1b . Figure 1: R-M and CRISPR1-Cas system cleave phage DNA. ( a ) Region of the phage 2972 genome analysed in this study. Each arrow represents an open reading frame (ORF) previously annotated [28] . The positions of protospacer S4 as well as HpaII restriction sites (5′-CCGG-3′) are indicated. ( b ) Zoom on a specific HpaII fragment of phage 2972 genome. LlaDCHI and DpnI restriction sites (5′-GATC-3′) are indicated. Details of expected cleaved and detected fragments by Southern hybridizations are given below, and the rectangle is a schematic representation of the probe used (5′-PS4) for hybridizations. ( c – e ) Southern hybridization of phage-infected S. thermophilus strains using wild-type phage 2972. Samples were taken after 5 min or after 15, 30 and 45 min intervals following the addition of phages. S. thermophilus strains DGCC7710+R-M, CRISPR-BIM S4, and BIM S4+R-M are represented by R-M, CRISPR-Cas (CR), and both respectively. The expected and detected cleaved DNA fragments are specified using different symbols (Δ, *, † and #). Five to ten micrograms of total DNA from DGCC7710 and CRISPR-BIM S4 were loaded per lane. All fragments belong to a different combination of CRISPR and/or R-M cleavage sites, but only the more important fragments implicating the CRISPR site are detailed in b . ( c ) Phage genome cleavage in S. thermophilus strains. The first panel to the left indicates the positive control (phage 2972 DNA). Specific cleavage activities detected in a : (i) R-M + strain (second panel; shorter fragment of ~1.2 kb), (ii) CRISPR-Cas strain (BIM S4, fourth panel; fragment of ~2.2 kb), (iii) strain carrying both an active R-M and CRISPR-Cas systems (third panel; shorter fragment of ~0.6 kb). ( d ) The 1.2-kb fragment obtained in c (second panel) in phage-infected S. thermophilus strain DGCC7710 carrying the LlaDCHI R-M system was followed over time (LlaDCHI; upper panel) in Southern hybridization assays. The same infected samples were restricted with DpnI, which cleaves only when its recognition site (5′-G m6 ATC-3′) is methylated (LlaDCHI+DpnI; lower panel). ( e ) The smaller fragment (0.6 kb) obtained in c (third panel) in phage-infected S. thermophilus strain DGCC7710 CRISPR-BIM S4 was followed over time. Only DpnI-restricted samples are shown as they give the same results as with LlaDCHI alone. Full size image Within 5 min after the beginning of the phage infection, several cleaved phage genomic fragments, including the shortest ~1.2-kb fragment, could be observed in DGCC7710 cells containing the R-M system ( Fig. 1c ), indicating that the endonuclease (R) has already digested the phage DNA at multiple GATC sites. Similarly, phage DNA was also cleaved, but as expected only once, within the protospacer region in the infected CRISPR-BIM S4 cells ( Fig. 1c , 2.2-kb fragment in CR lane). In cells containing the LlaDCHI R-M and an active CRISPR1-Cas system, phage DNA was cleaved by both mechanisms as shown by the observation of an ~0.6-kb fragment ( Fig. 1c , CR/R-M lane). While the restriction enzyme targets phage DNA as it enters the microbial cell, non-restricted phage DNA may also be modified by the R-M methylase [39] . Southern hybridizations using DNA extracts from a S. thermophilus RM-BIM strain infected by phage 2972 revealed that the amount of the 1.2-kb phage fragment was decreasing after 5 min, suggesting either its degradation or methylation of the flanking GATC sites over time (upper panel in Fig. 1d ). To discriminate between the above two hypotheses, we exploited the Dpn I recombinant enzyme, which specifically cleaves only methylated G m6 ATC sites as expected to be generated with the LlaDCHI system. We digested a portion of the extracted total DNA from phage-infected RM-BIM cells with DpnI before gel migration and Southern hybridization. The lower panel of Fig. 1d shows the presence of the phage genomic 1.2-kb fragment throughout the infection cycle, indicating that the phage DNA was indeed methylated in phage-infected R-M-containing cells. Of note, the 1.2-kb fragment in the lower panel of Fig. 1d contains the sum of methylated (showed by in vitro digestion of DpnI) and unmethylated ( in vivo digested by LlaDCHI) phage DNA, particularly evident at 5 min. Thus, as the phage infection proceeds over time, the unmethylated phage DNA is degraded and then, we observed only the methylated phage DNA, which increased over time (15–45 min). Taken together, this reveals that some restriction-resistant phages are produced and that they could propagate in a bacterial population harbouring only this R-M system. Using the same DpnI strategy as above, we checked the fate of the 1.2-kb phage fragment in a strain containing both the R-M and the CRISPR-Cas systems. Our results showed the appearance of a 0.6-kb fragment generated by the cleavage of the CRISPR-Cas system and the R-M system ( Fig. 1e ), which somehow appears to be degraded rapidly. Surprisingly, the 1.2-kb fragment persisted over time and may correspond to uncleaved CRISPR fragment as observed previously [26] and in Fig. 1c (fragment 3.1-kb). Impact of methylation The above results also suggested that the DNA cleavage activity of the CRISPR-Cas system may not be affected by the methylation provided by the LlaDCHI system. To confirm this, we further investigated the adenine methylation of the GATC recognition sites on the acquisition and interference activities of the CRISPR-Cas system. To do so, phage 2972 was propagated on the DGCC7710 host (without CR1-targeting spacer) containing LlaDCHI. While most of the phages were inactivated (EOP of 10 −5 ), some phages were able to multiply on this host. The genome of these phages was found to be methylated at the GATC sites as observed by their in vitro digestion by DpnI (the unmethylated genome of phage 2972 is not cleaved by DpnI) and by the in vivo phage replication (EOP of 1) on this strain. One methylated phage plaque was purified and amplified to high titers on LlaDCHI-containing cells. The fate of the GATC-methylated phage DNA was then followed as described in Fig. 1c during the infection of a CRISPR-BIM S4. The methylated phage DNA was cleaved by the CRISPR1 system within the protospacer region as expected (data not shown). These data were also correlated with the EOP of the methylated phage on the CRISPR-BIM S4, which was similar to the EOP of the non-methylated phage (10 −6 ). Because the protospacer S4 does not contain a GATC site, we selected additional CRISPR-BIMs (S57, S58 and S59) from our collection of natural mutants obtained in previous studies [12] , [13] , [27] that have acquired spacers containing a GATC restriction site (see Table 3 and Table 4 for spacer sequences and GATC positions). Then, we introduced the LlaDCHI system into them and the EOPs of phage 2972 were found to be similar to the BIM S4-containing pSRQ707 ( Table 1 ). EOPs of the methylated phage 2972 on these strains were also similar to those obtained on BIM S4 ( Table 5 ), confirming that this adenine methylation within these protospacers had no effect on the interference activity of the CRISPR-Cas system. Table 4 Characteristics of spacers acquired by BIMs used in this study. Full size table Table 5 Comparison of phage titers on a CR + -strain with or without the methylation conservation. Full size table While the CRISPR interference activity was not impaired by the adenine methylation in the GATC recognition sites, we also verified whether methylated phage DNA could limit spacer acquisition activity. Methylated phages were used to infect the S. thermophilus cells containing the R-M strain and BIMs were obtained as described elsewhere [12] . The CRISPR loci analysis of 80 randomly selected BIMs revealed that some of the newly acquired spacers contained a GATC recognition site, suggesting that the presence of a methylated DNA does not prevent spacer acquisition. The abundance of phages in virtually all bacteria-filled ecosystems has led to studies to try to understand this seemingly endless battle. A number of bacterial defence mechanisms and counterattacks by the phages were then uncovered. These dynamic evolutionary interactions help maintaining the phage–host balance in these environments [3] . R-M systems were discovered as a phage defence mechanism in early 1950s [5] and they were extensively leveraged in the next decades, which led to a revolution in genetic engineering. The phage resistance phenotype of CRISPR-Cas systems was observed 50 years later [13] and is apparently rapidly following in the same footsteps [14] , [18] , [19] . In their biological context, each DNA cleavage system provides significant protection to the microbial cell against invasion of foreign dsDNA, including phage genomes. However, they are also leaky on their own as phages can bypass these systems through a variety of means [3] , including the recently described anti-CRISPR phage genes [40] . While these phage responses might be perceived as a breach in the microbial arsenal, it should be reminded that these defence systems rarely work alone in a cell [3] . Here, we show that a type II CRISPR-Cas immune system can be compatible with a type II R-M systems to increase the overall phage resistance of bacteria. Each system can successfully cleave the dsDNA at their respective targeted sites in the presence of the other defence mechanism. The possibility of methylation as investigated here does not limit the main activities of the type II CRISPR-Cas system (adaptation and interference). It is believed that the combined action of both systems will considerably reduces the likelihood of emergence of phage derivatives capable of simultaneously evading R-M and CRISPR-Cas systems. It remains to be seen whether other types of CRISPR-Cas and R-M systems as well as other antiphage mechanisms will have similar additive protection. Bacterial strains, phages, plasmids and culture conditions S. thermophilus wild-type strain DGCC7710 and its derivatives ( Table 3 ) were grown at 37 °C or 42 °C in M17 broth supplemented with 0.5% lactose (LM17). The phage-resistant strain S. thermophilus BIM S4 is described elsewhere [12] , [26] . Plasmid pSRQ707 is a pNZ123-derivative vector containing the L. lactis LlaDCHI type II R-M system [34] , which was previously demonstrated to confer phage resistance in S. thermophilus strains [35] . LlaDCHI is an isoschizomer of MboI and DpnII (recognition sequence 5′-GATC-3′). This vector was introduced into various S. thermophilus strains by electroporation following a protocol already described [41] and using 1 μg of plasmid DNA and 40 μl of electrocompetent cells. Virulent phage 2972 (ref. 28 ) was routinely propagated on the wild-type S. thermophilus DGCC7710 strain in LM17 supplemented with 10 mM calcium chloride, at 42 °C. Phage 2972 containing methylated G m6 ATC sites was obtained after propagation on the strain DGCC7710 carrying the plasmid pSRQ707. High-titer phage preparations were obtained using polyethylene glycol [42] . When needed, phage 2972 was further purified by ultracentrifugation using a CsCl gradient [42] . Microbiological assays Unless specified otherwise, all microbiological assays were performed at 42 °C and S. thermophilus strains were grown to an optical density at 600 nm (OD 600 ) of 0.6. To measure the effect of CRISPR-Cas and R-M systems on phage resistance, the efficiencies of plaquing (EOPs) were determined by dividing the phage titer obtained by plating on a resistant strain by the titer of the same phage plated on the sensitive wild-type strain. Isolation of BIMs of S. thermophilus DGCC7710 BIMs (bacteriophage-insensitive mutants) were obtained by challenging phage-sensitive S. thermophilus strains with virulent phage 2972 (refs 28 , 43 ) as described elsewhere [12] . The four known CRISPR loci of S . thermophilus DGCC7710 and derivatives were analysed by PCR to determine the number of repeat-spacer units [12] , [25] , [26] , and by sequencing to obtain the spacer sequences. Primers used to perform PCR reactions are listed in the Table 6 . Table 6 Primers used in this study. Full size table Effect of phage methylation on the CRISPR-Cas system efficacy EOPs using the methylated phage lysate were evaluated on different BIMs to verify if the methylation of phage DNA changed CRISPR-interfering activity. EOPs of phage titers were calculated by dividing the phage titer obtained on a BIM with the titer obtained on the phage-sensitive wild-type strain. Moreover, some of the selected S. thermophilus BIMs (BIM S57, S58 and S59) contain a newly acquired spacer with a 5′-GATC-3′ LlaDCHI recognition site in their newly acquired 30-bp spacer. The other selected BIM (BIM S4) does not possess this recognition site in its new spacer. New BIM spacers and positions of the GATC sites are detailed in Table 4 . DNA cleavage by CRISPR-Cas and R-M during phage infection To determine the DNA cleavage activity for both systems, phage infections, subsequent DNA extraction and Southern blot assays were done as described previously [26] . Primer used to generate the Southern probes are detailed in Table 7 . S. thermophilus strains containing only one or both systems were analysed independently. Different time points during phage infection were selected to observe DNA cleavage over time. Infections were done by adding phages at a multiplicity of infection of at least 5 to exponentially growing cells (OD 600 of 0.6). For each sample, 5–10 μg of total DNA (coming from both phage and bacterial genomes) were loaded per lane. Table 7 Probe used for Southern blot assays. Full size table To observe the in vivo cleaved fragment by the CRISPR-Cas system, total phage-infected cell DNA was digested in vitro with HpaII (5′-CCGG-3′ sites) before Southern hybridization. The HpaII fragment of interest contains the phage 2972 protospacer region targeted by the probe and five LlaDCHI restriction sites (5′-GATC-3′) ( Fig. 1 ). LlaDCHI restriction endonuclease cleaved only non-methylated sites. In parallel, DpnI was used to detect G m6 ATC sites to determine if phage DNA molecules have been methylated over time by the LlaDCHI system. How to cite this article: Dupuis, M.-È. et al. CRISPR-Cas and restriction–modification systems are compatible and increase phage resistance. Nat. Commun. 4:2087 doi: 10.1038/ncomms3087 (2013).